Bioinspired desaturation of alcohols enabled by photoredox proton-coupled electron transfer and cobalt dual catalysis In the biosynthesis sterols an enzyme-catalyzed demethylation is achieved via a stepwise oxidative transformation of alcohols to olefins. The overall demethylation proceeds through two sequential monooxygenation reactions and a subsequent dehydroformylative saturation. To mimic the desaturation processes observed in nature, we have successfully integrated photoredox proton-coupled electron transfer (PCET) and cobaloxime chemistry for the acceptorless dehydrogenation of alcohols. The state-of-the-art remote and precise desaturation of ketones proceeds efficiently through the activation of cyclic alcohols using bond-dissociation free energy (BDFE) as thermodynamic driving force. The resulting transient alkoxyl radical allows C-C bond scission to generate the carbon-centered radical remote to the carbonyl moiety. This key intermediate is subsequently combined with cobaloxime photochemistry to furnish the alkene. Moreover, the mild protocol can be extended to desaturation of linear alcohols as well as aromatic hydrocarbons. Application to bioactive molecules and natural product derivatives is also presented. In the biosynthesis of sterols, a central reaction is the enzyme-catalyzed demethylation that involves a stepwise oxidative transformation of alcohols to olefins [1] , [2] , [3] , [4] . To trigger the C–C bond cleavage, the generation of an alkoxyl radical is believed to be crucial (Fig. 1a ). Inspired by this intriguing enzymatic process, we sought an analogous methodology for desaturation of alcohols in organic synthesis. The access of alkoxyl radicals via hydrogen atom transfer from the hydroxyl groups of aliphatic alcohols is straightforward but remarkably challenging. This is mainly attributed to the intrinsic difficulty of activating the kinetically inert O–H bonds [5] . In recent years, visible light photoredox catalysis has emerged as a powerful technique in organic synthesis that relies upon energetic electron transfer processes to facilitate previously thermally inaccessible or kinetically inert transformations [6] , [7] , [8] , [9] , [10] . In this context, the activation of O–H bonds has found broad utility in a number of reactions for the construction of C–C [11] , [12] , [13] , [14] , [15] , [16] , C–N [17] , [18] , [19] , C–S [20] , and C–X [21] , [22] bonds (Fig. 1b ). Despite these efforts, it is surprising to consider that the bioinspired olefin synthesis through acceptorless desaturation of alcohols remains an unmet challenge, to the best of our knowledge [23] . Fig. 1: Our inspiration from nature and previous work. a 14α-Demethylase ( CYP51 )-catalyzed demethylation of lanosterol and possible reaction mechanism. The CYP51 belongs to the family of cytochrome P450 enzymes. The demethylation proceeds through two sequential monooxygenation reactions and subsequently a dehydroformylation. b Ring-opening and functionalization of cycloalkanols enabled by photoredox catalysis. c Possible mechanism for stearoyl Δ9 desaturation. d Recent notable work on dehydrogenation via photoredox cobaloxime dual catalysis. e Desaturation of alcohols and aliphatic C–H bond via PCET/cobaloxime dual catalysis. Full size image Unsaturated carbonyl compounds are not only versatile synthetic building blocks, but also ubiquitous in natural products and biologically relevant molecules [24] , [25] , [26] , [27] , [28] , [29] . Although protocols for carbonyl desaturation at the adjacent sites (α-/β-) have been widely established, a mild and general strategy for remote site desaturation of ketone would be very appealing, but has not been reported. In nature, desaturase enzyme fascinates us with the regio- and stereoselective olefinic bond formation during the biosynthesis of fatty acid (Fig. 1c ) [30] . Notably, Baran [31] and Gevorgyan [32] , [33] recently reported auxiliaries assisted remote desaturation of alcohols and amines, through TEMPO mediated process or palladium photoredox catalysis, respectively. Given state-of-the-art remote functionalization, we considered that it is highly desirable to exploit readily accessible reaction partners with efficient catalyst systems to produce unsaturated ketones that are difficult to synthesize via conventional pathways. Recently, our group established a dual Nickel photoredox catalysis reaction to enable the remote cross coupling of tertiary alcohols [16] . This catalytic manifold provides a general and facile access to carbon-centered radicals remote to the carbonyl moiety via multiple site proton-coupled electron transfer (PCET) [34] , [35] . In line with the insight gained from this dual catalytic system, as well as recent developments on the dehydrogenative functionalization [36] , [37] , [38] , [39] , [40] , [41] , we envisioned the alkyl radical generated in this manner could in principle be merged with metallaphotoredox to realize the bioinspired acceptorless desaturation of alcohols. Enlighted by the most recent development on cobaloxime-based photoredox catalysis by Ritter, Sorensen and Leonori groups (Fig. 1d ) [42] , [43] , [44] , [45] , [46] , [47] , [48] , [49] , [50] , [51] , [52] , [53] , [54] , [55] , we became interested in the combination of photoredox PCET with the proton reduction reactivity of cobaloximes (Fig. 1e ). Here, we describe the development of a bioinspired acceptorless remote desaturation of tertiary, as well as secondary alcohols, via the photoredox PCET and cobalt synergistic catalysis and the extension to the desaturation to aromatic hydrocarbons, as well as silyl enol ethers. Rational design Our mechanistic proposal is shown in Fig. 2 . Upon visible light irradiation, a single electron transfer from the cyclohexanol derivative ( E p/2 = 1.57 V vs. SCE) [16] to the highly oxidizing singlet excited state * Mes – Acr – Me + ( E 1/2 red = +2.06 V vs. SCE) [6] would generate the corresponding arene radical cation along with the reduced form of the photocatalyst Mes – Acr – Me •. Subsequent multiple site PCET reaction between the hydroxyl group and the radical cation in the presence of base would give the key alkoxyl radical species, which readily cleaves into a carbonyl moiety and a distal carbon-centered radical through β scission of the neighboring C–C bond. The C-centered radical would subsequently be intercepted by the Co II species ( I ) to yield an alkyl–Co III intermediate ( II ), which can undergo C-cobalt bond homolysis upon light irradiation. Next, a, β-hydrogen abstraction by Co II at this stage would deliver the desired olefin and a cobalt III hydride species ( III ). Hydrogen gas evolves through the interaction between ( III ) and a proton generated in the PCET step. The cobalt and photoredox catalytic cycles then simultaneously complete via a single electron transfer event between Co III intermediate ( IV ) ( E 1/2 red = –0.68 V vs. SCE) and reduced form of photocatalyst C [56] , [57] . Fig. 2: Our envisioned mechanism proposal. Photoredox PCET/cobaloxime dual catalysis enabled desaturation of alcohols. PMP p -methoxy phenyl group. 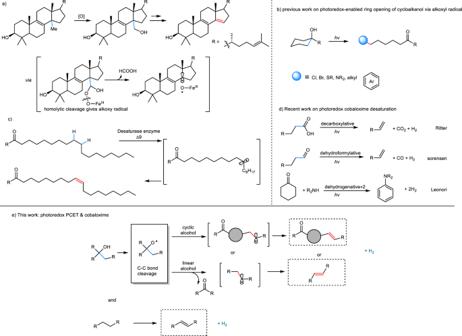Fig. 1: Our inspiration from nature and previous work. a14α-Demethylase (CYP51)-catalyzed demethylation of lanosterol and possible reaction mechanism. TheCYP51belongs to the family of cytochrome P450 enzymes. The demethylation proceeds through two sequential monooxygenation reactions and subsequently a dehydroformylation.bRing-opening and functionalization of cycloalkanols enabled by photoredox catalysis.cPossible mechanism for stearoyl Δ9 desaturation.dRecent notable work on dehydrogenation via photoredox cobaloxime dual catalysis.eDesaturation of alcohols and aliphatic C–H bond via PCET/cobaloxime dual catalysis. Full size image Optimization of the reaction conditions The reaction conditions optimization of the synergistic combination of photoredox and cobalt catalysis is briefly summarized in Table 1 . The initial evaluation focused on readily available substrate 1a to mimic the enzymatic process, namely Δ9 desaturation of stearoyl-CoA (Fig. 1c ). Optimized reaction conditions were readily established, using 7.5 mol% PC - I Mes–Acr–Me + , 10 mol% Co(dmgH) 2 (py) 2 PF 6 and 2 equiv. 2,4,6-collidine in a 0.1 M solution of 1,2-dichloroethane (DCE) at room temperature with blue light-emitting diodes (LEDs) irradiation. Under these conditions, the desired product was formed in 93% NMR yield and very good selectivity (22:1) (Table 1 , entry 1). Use of less oxidizing photosensitizers such as [Ru(bpy) 3 ](PF 6 ) 2 ( PC - II , E 1/2 [Ru *III /Ru II = + 0.77 V vs. SCE in CH 3 CN]) [58] and [Ir(dF(CF 3 )ppy) 2 (bpy)]PF 6 ( PC - III , E 1/2 [Ir *III /Ir II = + 1.21 V vs. SCE in CH 3 CN]) [59] resulted in no product or trace amounts of product, while the strong oxidizing [Ir(dF(CF 3 )ppy) 2 (5,5’(CF 3 )bpy)]PF 6 ( PC - IV , E 1/2 [Ir *III /Ir II = + 1.68 V vs. SCE in CH 3 CN]) gave 2a in 71% yield (entries 2 to 4). A screening of different organic and inorganic bases revealed that collidine was the best choice (entries 5 and 6). 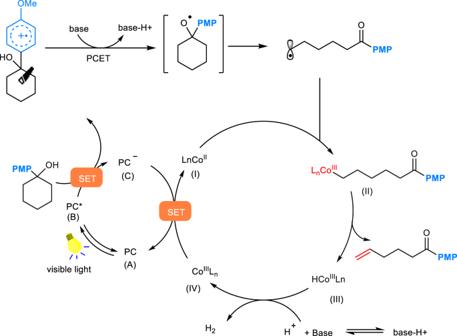Fig. 2: Our envisioned mechanism proposal. Photoredox PCET/cobaloxime dual catalysis enabled desaturation of alcohols. PMPp-methoxy phenyl group. The use of Co(dmgH)(dmgH 2 )Cl 2 and Co(dmgH) 2 PyCl as cobaloxime sources leads to a decrease of yields and selectivities (entries 7 and 8). When the reaction was conducted in HFIP or MeCN, the amount of product could be negligible. The reaction efficiency diminished dramatically when toluene was employed, while a comparable result was observed using DCM (entries 9–12). The inverse relationship between solvent polarity and yield can be taken as support for the intermediacy of hydrogen bonding, because the polar interaction is generally disfavored in polar solvent. It is not surprising to observe that control experiments performed without photocatalyst, Co catalyst, base or light each failed to give any desired product (Table 1 , entry 13). Table 1 Optimization of the reaction conditions a,b . Full size table Substrate scope As illustrated in Fig. 3 , we found the desaturation protocol was tolerant to a wide range of alcohols and gave the corresponding olefinic products in moderate to very good yields. To begin with, it was found that cyclic tertiary alcohols with different ring sizes ( 1a – 1h ) all reacted smoothly to selectively generate remote desaturated ketones regardless of their ring strains ( 2a – h , 51–91% yields). Notably, due to the base mediated isomerization, the α-/β-sites desaturation product was obtained exclusively with prolonged reaction time in the reaction of cyclobutanol 1b . Symmetrical substituted cyclohexanols ( 1i to 1p ) behaved well to give products 2i to 2p in moderate yields (42–68%). Functional groups including trifluoromethyl, silyl ether, geminal difluoride, nitrile and amide could be well tolerated. The ring-opening of unsymmetrical cyclohexanols 1r and 1s took place regioselectively and, the remarkable selectivity can be explained by C–C bond cleavage favors the formation of more stabilized carbon-centered radical ( 2r and 2s , 60% and 82% yields). Fig. 3: Scope of cyclic and linear alcohols. General reaction conditions: 1 (1 equiv. ), 2,4,6-collidine (2 equiv. ), PC - I (7.5 mol%), Co(dmgH) 2 (py) 2 PF 6 (10 mol%), DCE (0.1 M), rt, blue LEDs, 48–72 h. a 1 or 3 mol% [Ir(dF(CF 3 )ppy) 2 (5,5′d(CF 3 )bpy)](PF 6 ) PC-IV was used. b NBu 4 OP(O)(OPh) 2 as base. 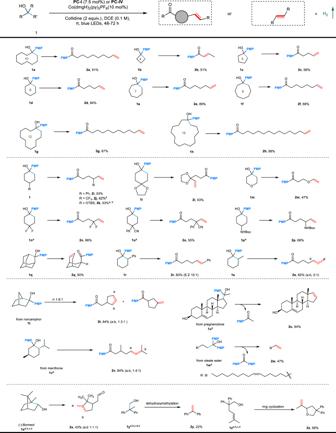Fig. 3: Scope of cyclic and linear alcohols. General reaction conditions:1(1 equiv.), 2,4,6-collidine (2 equiv.),PC-I(7.5 mol%), Co(dmgH)2(py)2PF6(10 mol%), DCE (0.1 M), rt, blue LEDs, 48–72 h.a1 or 3 mol% [Ir(dF(CF3)ppy)2(5,5′d(CF3)bpy)](PF6)PC-IVwas used.bNBu4OP(O)(OPh)2as base.cToluene or PhCF3as solvent.d5 mol% Co catalyst was used in2uto2z.e1H NMR yield with internal standard. c Toluene or PhCF 3 as solvent. d 5 mol% Co catalyst was used in 2u to 2z . e 1 H NMR yield with internal standard. Full size image For the norcamphor-derived bridged bicyclic substrate 1t , mixture of isomers was observed as a result of poor selectivity in the ring-opening. In contrast, a menthone derivative displays excellent regioselectivity in the ring-opening step ( 1v , 84%). Moreover, we successfully extended the scope to linear tertiary alcohols derived from pregnenolone and oleate ester, affording the corresponding olefins 2u and 2w in moderate to excellent yields. In addition to tertiary alcohols, naturally occurring secondary alcohol 1x proved to be competent substrate for the PCET enabled regioselective ring-opening/desaturation sequence. Remarkably, the dehydroxymethylative desaturation of 2,2-diphenylpropan-1-ol could take place, affording the diphenylethylene in 22% yield. Next, we found that the cascade ring cyclization/desaturation was feasible, a moderate yield of cyclized product was obtained ( 2z , 56%). With the above success, we next examined the generality of the photoredox-cobalt desaturation with respect to the arene substituent on the cyclic ring. As shown in Fig. 4 , a variety of arene-substituted cyclohexanols performed well. Monosubstituted aromatics such as tert -butyl–, phenyl–, and tert -butyldimethylsilyl (TBS)-protected phenols as well as biphenyl are suitable candidates ( 4a – 4d , 58–74% yields). Disubstituted anisole derivative was also suitable substrate for this transformation ( 4e , 72% yield). Both naphthalene- and phenanthrene-substituted cyclohexanols smoothly underwent ring-opening/desaturation under these conditions ( 4f and 4g , 52% and 47% yields). Interestingly, minor amount of α-/β-sites desaturation product was obtained in the case of 4f , this can be accounted for by Co III -hydride mediated chain walking process [51] . Following the success, privileged heteroaromatics including benzofuran and thiobenzofuran could also be used ( 4h and 4i , 43% and 63% yields). Fig. 4: Scope of arene substituents. Reaction conditions: 3 (0.2 mmol, 1 equiv. ), 2,4,6-collidine (0.4 mmol, 2 equiv. ), PC - I (7.5 mol%), Co(dmgH) 2 (py) 2 PF 6 (10 mol%), DCE (2.0 mL, 0.1 M), rt, blue LEDs, 48–72 h. Full size image To further highlight the robustness of this protocol, tetrahydronaphthalene 5a was subjected to the reaction conditions (Fig. 5 ). The desaturation takes place selectively to release 2 molar equiv. hydrogen gas and no dihydronaphthalene product was observed, indicating the second desaturation should be easier than the initial one. Therefore, two styrene derivatives were examined next, to give products such as 6b and 6c in good to excellent yields. Heterocycle such as 6d can also be prepared in good yield (74%). Moreover, when benzylic alcohols were employed in the PCET enabled acceptorless desaturation, the corresponding aldehyde and ketone products were obtained in excellent yields ( 6e and 6f ). Importantly, this protocol was able to transform silyl enol ethers into silyloxyarenes in moderate to good yields [60] . For example, desaturation of 5g leads to the formation of tert -butyl(dimethyl)silyl (TBS) ether of α-naphthol with excellent efficiency ( 6g , 84% yield). Silyl enol ethers derived from cyclohexanones were also amenable to the current protocol via the removal of two molecules of hydrogen gas, with no detection of α, β-desaturated ketone product ( 6h and 6i , 51% and 72% yields, respectively). This intriguing selectivity stands in stark contrast to previous dehydrogenation reactions that exclusively affording cyclohexenones [61] , [62] . Fig. 5: Scope of aromatic hydrocarbons and silyl enol ether. Reaction conditions: 5 (0.2 mmol, 1 equiv. ), 2,4,6-collidine (0.2 mmol, 1 equiv. ), [Ir(dF(CF 3 )ppy) 2 (5,5′d(CF 3 )bpy)](PF 6 ) PC-IV (1 mol%), Co(dmgH) 2 (py) 2 PF 6 (10 mol%), DCE (1.0 mL, 0.2 M), rt, blue LEDs, 36 h. Full size image Next, we carried out the synthesis of remote unsaturated ketone 2a on a preparative scale (2 mmol) under our optimal conditions, providing the expected olefinic product 1a in 81% yield (Fig. 6a ). To showcase the synthetic utility of the product provided by this methodology, 2a was converted efficiently to a fatty acid ester epoxide during a Baeyer-Villiger oxidation (Fig. 6b ). Following a Grignard reaction of 2a , the linear product 8 was subjected further to the reaction conditions, an interesting diene 9 was isolated in 51% yield (Fig. 6c ). Fig. 6: Scale up and synthetic utility. a Reaction on large scale, under standard conditions: tertiary alcohol (1 equiv. ), 2,4,6-collidine (2 equiv. ), PCI (7.5 mol%), Co(dmgH) 2 (py) 2 PF 6 (10 mol%), DCE (0.1 M), rt, blue LEDs, 48 h. b Baeyer-villiger oxidation. c sequential desaturation to synthesize diene. Full size image Apart from the control experiments shown in Table 1 , we conducted some preliminary mechanistic experiments to gain some insight of the metallaphotoredox desaturation protocol. When the reaction mixture was subjected to a radical scavenger 2,2,6,6-Tetramethyl-1-piperidinyloxy (TEMPO, 1 equiv.) under the standard conditions, no product was detected. A remote TEMPO-trapped ketone 10 was instead formed, implying that a radical process is involved in the catalytic cycle (Fig. 7a ). The generation of carbon-centered radical remote to the carbonyl group was further supported by the Heck-Type coupling with styrene, affording 11 (Fig. 7b ). To gain more insight into the reaction, the formation of molecular hydrogen was quantitatively analyzed by gas chromatography. Importantly, we observed that more than 1 equiv. hydrogen gas was produced with substrate 5a , in contrast the generation of H 2 is less than 1 equiv. in the case of 1d . The kinetic profile of H 2 evolution of substrate 1d shows a fast gas production rate in the first hours, however, it becomes very sluggish after 6 h (Fig. 7c, d ). This result is consistent with our observation that the desaturation of alcohols generally required long reaction time, we assume that the increasing amount of free base has a marked effect on the hydrogen production [63] . Fig. 7: Preliminary experiments on the reaction mechanism. a Radical-trapping experiment with free-radical scavenger. b Heck-Type coupling with styrene. c Reaction conditions and results for H 2 production of substrates 1d and 5a . d H 2 production rate monitoring and quantification for substrates 1d and 5a . Full size image In conclusion, we have developed a bioinspired acceptorless desaturation of tertiary as well as secondary alcohols via the photoredox PCET and cobalt synergistic catalysis. The manifold provides a concise access to remotely dehydrogenated ketones that are difficult to synthesize with current methods, through ring-opening/desaturation of cyclic alcohols. We also demonstrated the strategy could be applied to linear alcohol, aromatic hydrocarbons as well as silyl enol ethers. 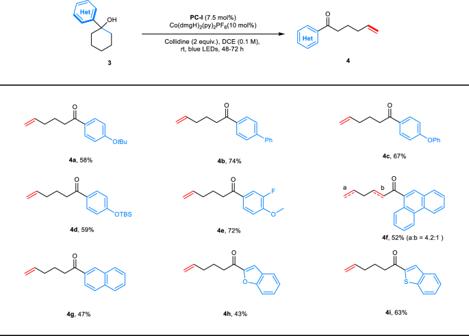Fig. 4: Scope of arene substituents. Reaction conditions:3(0.2 mmol, 1 equiv.), 2,4,6-collidine (0.4 mmol, 2 equiv.),PC-I(7.5 mol%), Co(dmgH)2(py)2PF6(10 mol%), DCE (2.0 mL, 0.1 M), rt, blue LEDs, 48–72 h. Importantly, a variety of bioactive molecules and natural product derivatives were all well tolerated under such mild conditions. In consideration with numerous findings about the essential role of PCET in biological redox processes, this contribution expands the less-developed applications of PCET in organic synthesis. General procedure for bioinspired dehydrogenation of alcohols To a 15 mL vial equipped with a stir bar was added Co(dmgH) 2 (py) 2 PF 6 (12 mg, 0.02 mmol, 10 mol%), and photocatalyst (9-mesityl-10-methylacridinium perchlorate 7.5 mol% or [Ir(dF(CF 3 )ppy) 2 (5,5′d(CF 3 )bpy)](PF 6 ) 1 mol%), collidine (1 or 2 equiv.) and tertiary alcohol (0.2 mmol, 1 equiv.). The vial was sealed, evacuated and backfilled with Argon three times, then 2 mL of DCE was added. After degassing with Freeze–Pump–Thaw methods for three cycles, it was stirred and irradiated with the corresponding blue LEDs photoreactor. 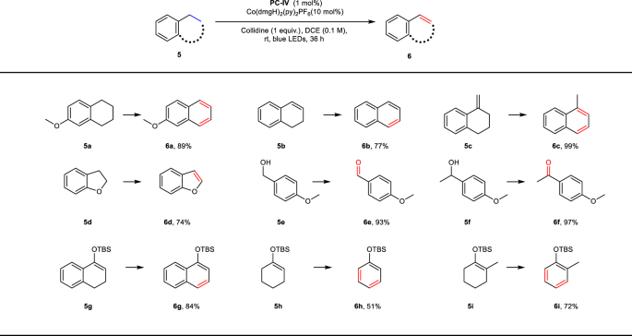Fig. 5: Scope of aromatic hydrocarbons and silyl enol ether. Reaction conditions:5(0.2 mmol, 1 equiv.), 2,4,6-collidine (0.2 mmol, 1 equiv.), [Ir(dF(CF3)ppy)2(5,5′d(CF3)bpy)](PF6)PC-IV(1 mol%), Co(dmgH)2(py)2PF6(10 mol%), DCE (1.0 mL, 0.2 M), rt, blue LEDs, 36 h. 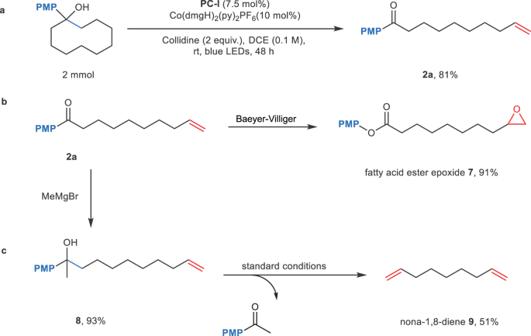Fig. 6: Scale up and synthetic utility. aReaction on large scale, under standard conditions: tertiary alcohol (1 equiv.), 2,4,6-collidine (2 equiv.),PCI(7.5 mol%), Co(dmgH)2(py)2PF6(10 mol%), DCE (0.1 M), rt, blue LEDs, 48 h.bBaeyer-villiger oxidation.csequential desaturation to synthesize diene. 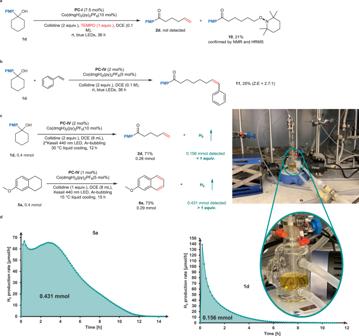Fig. 7: Preliminary experiments on the reaction mechanism. aRadical-trapping experiment with free-radical scavenger.bHeck-Type coupling with styrene.cReaction conditions and results for H2production of substrates1dand5a.dH2production rate monitoring and quantification for substrates1dand5a. Upon completion, the reaction mixture was concentrated in vacuo and purified with column chromatography to afford the desired product.